Direct observation of two-electron Ag(I)/Ag(III) redox cycles in coupling catalysis Silver is extensively used in homogeneous catalysis for organic synthesis owing to its Lewis acidity, and as a powerful one-electron oxidant. However, two-electron redox catalytic cycles, which are most common in noble metal organometallic reactivity, have never been considered. Here we show that a Ag(I)/Ag(III) catalytic cycle is operative in model C–O and C–C cross-coupling reactions. An aryl-Ag(III) species is unequivocally identified as an intermediate in the catalytic cycle and we provide direct evidence of aryl halide oxidative addition and C–N, C–O, C–S, C–C and C–halide bond-forming reductive elimination steps at monometallic silver centres. We anticipate our study as the starting point for expanding Ag(I)/Ag(III) redox chemistry into new methodologies for organic synthesis, resembling well-known copper or palladium cross-coupling catalysis. Furthermore, findings described herein provide unique fundamental mechanistic understanding on Ag-catalysed cross-coupling reactions and dismiss the generally accepted conception that silver redox chemistry can only arise from one-electron processes. Organic chemistry has taken advantage of the catalytic transformations promoted by most transition metals, although some of them, such as silver, have only gained interest in the past few years. Silver holds the most unexplored chemistry among the coinage metals and its redox chemistry is the least understood [1] , [2] , [3] , [4] , [5] . Ag(I) salts are commonly employed in organic transformations by exploiting three main properties ( Fig. 1 ). First, its moderate Lewis acidity has found application in activating allenes and alkynes to promote a nucleophilic attack over the unsaturation to render, for instance, the cyclization of allenols, allenones and allenoic acids [4] , [5] . The π-activation of terminal acetylenes can also produce silver(I)-acetylides [6] , [7] , which are known as efficient transmetallating agents and have been widely utilized in organopalladium catalysis [8] , [9] , [10] . The second important characteristic of Ag(I) chemistry is the insolubility of its corresponding halide salts (halogenophilicity). A large number of transition metal-catalysed reactions are conducted in the presence of Ag(I) salts to trigger the precipitation of Ag X salts ( X =Cl, Br, I) from coordinatively saturated metal centres, for instance, in Pd-catalysed cross-coupling reactions involving aryl or alkenyl halides [5] , or in Au-catalysed C–C bond-forming reactions [11] . Finally, Ag(I) salts are extensively used as one-electron oxidant, for instance in the preparation of carbonyls from the corresponding alcohols under mild conditions [2] , [12] . More recently, an increasing number of oxidative C–C bond-forming reactions of arenes require the use of a sacrificial outer-sphere oxidant, and Ag(I) is often the oxidant of choice [13] . 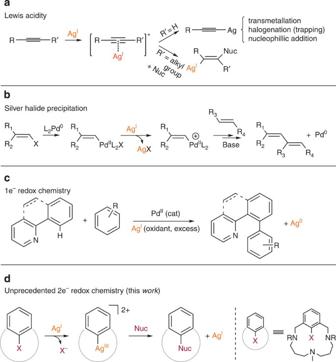Figure 1: Canonical reactivity of silver. (a) Activation of C–C insaturations due to its Lewis acid character. (b) Halogenophilicity to drive reactions by forming insoluble halide salts (AgX). (c) Use as sacrificial oxidant by promoting the one-electron oxidation of the metal catalyst. (d) Novel two-electron-based reactivity described in this work involving Ag(I)/Ag(III) redox processes. Figure 1: Canonical reactivity of silver. ( a ) Activation of C–C insaturations due to its Lewis acid character. ( b ) Halogenophilicity to drive reactions by forming insoluble halide salts (AgX). ( c ) Use as sacrificial oxidant by promoting the one-electron oxidation of the metal catalyst. ( d ) Novel two-electron-based reactivity described in this work involving Ag(I)/Ag(III) redox processes. Full size image It is generally accepted that silver involves exclusively one-electron redox chemistry [4] , [14] , [15] , [16] , [17] , in contrast to the other two group-11 metals, copper and gold, which can undergo two-electron redox chemistry. Copper and gold have been directly implicated in M(I)/M(III) oxidative addition and reductive elimination processes [18] , [19] , [20] , [21] , [22] , [23] , [24] , [25] , whereas such chemistry has never been considered for silver. Nevertheless, silver has been reported as an effective catalyst in cross-coupling reactions such as Ag-catalysed Sonogashira couplings [26] and Ag-catalysed Ullmann-type C-heteroatom bond-forming reactions [27] . However, no mechanistic studies have been carried out so far to rationalize these transformations. Ritter and co-workers proposed recently the presence of bimetallic aryl-Ag(II)-Ag(II)-F species in silver(I)-mediated electrophilic fluorination of aryl stannanes [14] . Instead, Li and co-workers suggest in their studies on Ag(I)-catalysed radical aminofluorinations that electrophilic fluoride sources are capable of generating monometallic Ag(III)-F intermediate species [28] , although the C–F bond formation is proposed to occur through reaction of a Ag(II)-F and a carbon-centred radical species, following a one-electron redox sequence. No direct evidence of the intermediates proposed is reported, thus mechanistic comprehension of silver-catalysed processes stands as its Achilles heel for future design of new synthetic methodologies. Herein we report the discovery that silver can be engaged in two-electron oxidative addition and reductive elimination processes and that, indeed, a Ag(I)/Ag(III) catalytic cycle is operative in model C-O and C-C cross-coupling reactions ( Fig. 1d ). We provide direct spectroscopic and crystallographic characterization of a well-defined aryl-Ag(III) species, which is identified as the catalytically active species. Synthesis and full characterization of the Ag(III) complex The synthesis of aryl-Ag(III) complex 1 ClO4 was achieved by reacting the model aryl-halide ligand L 1 -Br with 2 equiv. of Ag(I)ClO 4 , affording [Ag(III) L 1 ](ClO 4 ) 2 ( 1 ClO4 , 68% yield) and AgBr that precipitates from the solution ( Fig. 2a ). This complex is bench-top stable and has been fully characterized spectroscopically and crystallographically. The structure obtained by X-ray diffraction studies of compound 1 ClO4 shows that the Ag(III) centre is tetracoordinated and exhibits a nearly square planar geometry, in which the aryl moiety and three amine N atoms are coplanar with the silver centre ( Fig. 2b ). 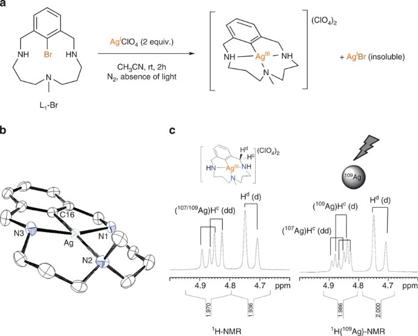Figure 2: Synthesis and characterization of the aryl-Ag(III) complex (1ClO4). (a) Synthesis of the aryl-Ag(III) species (1ClO4). (b) X-ray diffraction: thermal ellipsoid diagram (at 50% probability level) of the cationic moiety of1ClO4. The hydrogen atoms and the two perchlorate anions have been omitted for clarity. Selected bond lengths [Å] and angles [°] of1ClO4: Ag-C(16) 1.974(2), Ag-N(3) 2.084(2), Ag-N(1) 2.085(5), Ag-N(2) 2.153(2); C(16)-Ag-N(3) 82.03(10), C(16)-Ag-N(1) 81.6(1), N(3)-Ag-N(2) 98.2(1), N(1)-Ag-N(2) 98.4(1), C(16)-Ag-N(2) 178.2(1), N(3)-Ag-N(1) 162.1(1). (c) Comparison of the benzylic region of1ClO4in the1H NMR and1H{109Ag} NMR experiments (298 K, CD3CN, 400 MHz NMR; seeSupplementary Information). Figure 2: Synthesis and characterization of the aryl-Ag(III) complex ( 1 ClO4 ). ( a ) Synthesis of the aryl-Ag(III) species ( 1 ClO4 ). ( b ) X-ray diffraction: thermal ellipsoid diagram (at 50% probability level) of the cationic moiety of 1 ClO4 . The hydrogen atoms and the two perchlorate anions have been omitted for clarity. Selected bond lengths [Å] and angles [°] of 1 ClO4 : Ag-C(16) 1.974(2), Ag-N(3) 2.084(2), Ag-N(1) 2.085(5), Ag-N(2) 2.153(2); C(16)-Ag-N(3) 82.03(10), C(16)-Ag-N(1) 81.6(1), N(3)-Ag-N(2) 98.2(1), N(1)-Ag-N(2) 98.4(1), C(16)-Ag-N(2) 178.2(1), N(3)-Ag-N(1) 162.1(1). ( c ) Comparison of the benzylic region of 1 ClO4 in the 1 H NMR and 1 H{ 109 Ag} NMR experiments (298 K, CD 3 CN, 400 MHz NMR; see Supplementary Information ). Full size image The Ag–C bond length is 1.974 Å, the shortest in the silver coordination sphere of 1 ClO4 , and also among the scarce number of organometallic Ag(III) complexes reported in the literature [29] , [30] , [31] , [32] . The short Ag–C bond distance along with the charge balance of the complex, its diamagnetic nature and density functional theory (DFT) (B3LYP-D 2 /6-311+G**) spin densities indicate that the metal centre is best described as Ag(III). Indeed, 1 ClO4 is isostructural with the previously described and fully characterized aryl-Cu(III) complex [33] , [34] , and the DFT optimized geometry is also in agreement with the crystallographic characterization (see Supplementary Fig. 1 ). NMR studies ( 1 H-NMR and one-dimensional (1D) 109 Ag-decoupled 1 H-NMR, see Fig. 2c and Supplementary Figs 2–9 ) and high-resolution mass spectrometry (HRMS) analysis ([C 15 H 24 N 3 AgClO 4 ] + , m / z =454.0495; Supplementary Fig. 10 ) are conclusive to state that the aryl-Ag(III) maintains the same structure in solution than in the solid state. Moreover, a 1 H- 109 Ag heteronuclear multiple bond correlation (HMBC) experiment allowed the determination of the 109 Ag chemical shift (2,127 p.p.m. ), which is in close agreement to that reported for other Ag(III) complexes ( Supplementary Fig. 5 ) [32] . For further discussion on the NMR analysis of 1 ClO4 , see Supplementary Discussion 1 . Reactivity of the Ag(III) complex Once 1 ClO4 was fully characterized, we turned our attention towards its reactivity. We speculated that this complex could show a similar reactivity to its analogous copper complex, that is, to undergo reductive eliminations to functionalize the C sp2 - M (III) ( M =Cu or Ag) bond in the presence of nucleophiles of different nature [19] , [35] . The reaction of 1 ClO4 with sulfonamides, aromatic and aliphatic carboxylic acids, phenols and thiophenols resulted in the formation of C aryl –nucleophile coupling products in excellent yields, characteristic of a reductive elimination reaction (products 2a - 2g , Table 1 ). p -Thiocresol is the substrate that exhibits the fastest reactivity with the aryl-Ag(III) complex, reaching completion after only 1 min ( Table 1 , entry 7). Furthermore, NaCN also reacts with 1 ClO4 to form the C–C coupling product ( L 1 -CN , Table 1 , entry 8) in good yield. Strikingly, C–C coupling products were also obtained in excellent yields when malononitrile [36] and aryl boronic acids were used as coupling partners ( Table 1 , entries 9–11). The above reductive elimination processes rendered the C–nucleophile coupling products and Ag(I) species; the latter was detected by performing the reaction of 1 ClO4 with 1 equiv. of p -nitrophenol to full conversion and subsequently adding 3 equiv. of PPh 3 to form Ag(I)(PPh 3 ) n species. 31 P{ 1 H} NMR showed a broad doublet at 7.93 p.p.m. (J( 31 P- 109 Ag)=343 Hz), which exactly matched the signal observed in a sample prepared by reacting Ag(I)ClO 4 with 3 equiv. of PPh 3 ( Supplementary Figs 11 and 12 ). Moreover, these reactions were unaffected by the addition of TEMPO radical; this observation disfavours a radical-mediated process ( Table 1 , entry 4). To the best of our knowledge, these are the first examples of fully characterized two-electron reductive elimination processes from a well-defined Ag(III) complex. Table 1 Stoichiometric coupling of nucleophiles with 1 ClO4 complex*. Full size table We then explored the C–halide reductive elimination reaction by treating 1 ClO4 with 2 equiv. of nBu 4 N X ( X =I, Br, Cl) salts, and found that the corresponding L 1 –X coupling products were obtained quantitatively ( Table 1 , entries 12–14). Aryl fluorination was also attempted, affording a 39% yield of the desired fluorinated arene ( L 1 –F ) when the reaction was run in the presence of 2 equiv. of n Bu 4 NF·3H 2 O at 40 °C in acetonitrile ( Table 1 , entry 15). Detrimental deprotonation of 1 ClO4 by the basic fluoride anion was avoided by using the N -permethylated L 5 –Br aryl bromide model substrate, obtaining quantitative formation of L 5 –F product ( Fig. 3 ; see also Supplementary Figs 13–15 for additional information in fluorination reactions) [37] , [38] , [39] . DFT calculations show that the reductive elimination of L 5 –Ag(III) is strongly exergonic (ΔG=−25.8 kcal·mol −1 ) and has a very low barrier (ΔG ≠ =8.6 kcal·mol −1 ; for computed reaction profile see Supplementary Fig. 16 ). 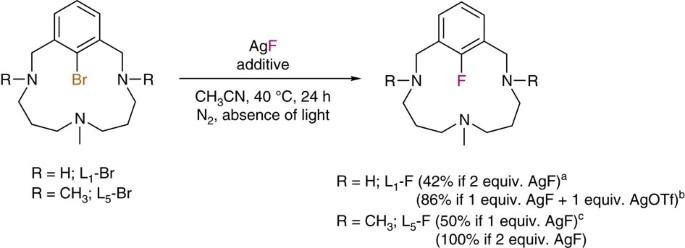Figure 3: Silver(I)-mediated fluorination of model aryl halide substrates. General conditions: model aryl halide (Ln–X) 12–14 μmol, AgF 12–28 μmol, AgOTf 0–12 μmol, 2 ml CH3CN, 40 °C. Yields calculated by1H-NMR spectroscopy using 1,3,5-trimethoxybenzene as internal standard.a13% of intramolecular C–N coupling product.39b8% of intramolecular C–N coupling product.39c20%L5–Br(remaining starting material). Figure 3: Silver(I)-mediated fluorination of model aryl halide substrates. General conditions: model aryl halide ( L n – X ) 12–14 μmol, AgF 12–28 μmol, AgOTf 0–12 μmol, 2 ml CH 3 CN, 40 °C. Yields calculated by 1 H-NMR spectroscopy using 1,3,5-trimethoxybenzene as internal standard. a 13% of intramolecular C–N coupling product. [39] b 8% of intramolecular C–N coupling product. [39] c 20% L 5 –Br (remaining starting material). Full size image Study of the Ag(III) complex synthesis Concerning the aryl halide oxidative addition step ( Supplementary Table 1 ), we found that for aryl-Br ( L 1 –Br ) and aryl-I ( L 1 –I ) model substrates, yields of 1 ClO4 were almost quantitative when 2 equiv. of AgOTf were used (25 °C). On the contrary, if only 1 equiv. of AgOTf was used, yields no higher than 50% were observed. We rationalized these results by considering that 1 equiv. of silver(I) loading is consumed to form the desired aryl-Ag(III) product, whereas the second Ag(I) equivalent traps the halide to precipitate as Ag X ( X =Br, I). However, a bimetallic centred process similar to Ritter’s proposal could not be ruled out at this point [14] . Addition of Tl(OTf) as an additive to directly compete for the formation of extremely insoluble thalium halide salts, afforded 1 OTf in 68% yield by using 1 equiv. of AgOTf, 1 equiv. of Tl(OTf) and L 1 -I , thus strongly supporting our monometallic oxidative addition proposal ( Supplementary Table 1 ). We additionally tested these reactions with L 1 –Cl as model substrate, but no aryl-Ag(III) product was observed. The DFT-computed reaction profiles for the oxidative addition of Ag(I) over L 1 –F , L 1 –Cl , L 1 –Br and L 1 –I show a decrease of the Gibbs energy barriers (Δ G ≠ ( L 1 – X )=33.2, 18.1, 14.4, 11.2 kcal·mol −1 for X =F, Cl, Br, I, respectively) and reaction Gibbs energies (Δ G ( L 1 – X )=17.6, 1.8, 0.8, −7.5 kcal·mol −1 for X =F, Cl, Br, I, respectively; for computed reaction profiles see Supplementary Fig. 17 ). The trends extracted from DFT calculations nicely agree with the observed formation of the Ag(III) complex with L 1 –Br and L 1 –I but not with L 1 –Cl and L 1 –F . Model C–O bond-forming cross-coupling reactions Provided that the fundamental details of two-electron Ag(I)/Ag(III) oxidative addition and reductive elimination redox steps were understood individually, we merged both steps in a single C-heteroatom cross-coupling reaction. We selected p -nitrophenol as the nucleophile to be reacted with L 1 – X ( X =I, Br, Cl) in the presence of 1 equiv. of AgOTf at 50 °C ( Table 2 ). The C–O coupling product 2d was obtained in 75% and 64% yield when L 1 –I and L 1 –Br were used, respectively ( Table 2 , entries 1, 10). In the case of L 1 –I , if a slight excess of AgOTf is used (1.1 equiv. ), a 95% yield of 2d is obtained ( Table 2 , entry 2). These results suggest that after initial oxidative addition, a 50% of the silver precipitates as AgI, whereas the other 50% produces Aryl-aryl-Ag(III) that reacts with the nucleophile and reductively eliminates the coupling product 2d , thus a 50% Ag(I) is set free again (assuming quantitative reductive elimination) to react again with more L 1 –I . The same reactivity pattern is repeated after each cycle with the remaining free Ag(I) in solution. However, we cannot exclude the potential beneficial effect of using excess of nucleophile (20 equiv.) as we have observed that it severely prevents the precipitation of AgI ( vide infra ). Moreover, when L 1 –Cl was used we could obtain a 37% yield of the desired product ( Table 2 , entry 13), thus in agreement with the computed kinetic feasibility of the oxidative addition of L 1 –Cl (Δ G ≠ =18.1 kcal·mol −1 ). Table 2 Silver-catalysed C–O and C–C bond-forming cross-coupling reaction with L 1 –X model substrates*. Full size table Catalytic cross-coupling reactions via silver(III) species The positive results for the C–O cross-coupling reactions stoichiometric in silver(I) prompted us to explore the catalytic version of these processes ( Table 2 ). The first attempts employing L 1 –I (1 equiv. ), p -nitrophenol (2 equiv.) and 10 mol% of AgOTf as the catalyst (in CH 3 CN, absence of light) failed to provide more than 1 catalytic cycle as only 9% of the desired biaryl ether product 2d was obtained ( Supplementary Table 2 ), along with a yellow precipitate. The undesired precipitation of catalytic silver as AgI was prevented by increasing the amount of nucleophile up to 20 equiv. and we observed that the C–O coupling product yield increased up to 37% ( Table 2 , entry 3). We optimized the reaction in the presence of phosphines with distinct electron donor strength to further stabilize the Ag(I) cations in solution ( Table 2 , Supplementary Discussion 2 and Supplementary Table 2 ). Among the auxiliary ligands tested, PPh 3 (10 mol%) was the best choice giving a 46% yield of the biaryl ether product 2d ( Table 2 , entry 4). We were pleased to find that a 74% yield of the desired product 2d was achieved by increasing the catalyst loading to 20 mol% and employing a 20 mol% of PPh 3 ( Table 2 , entry 5). Under the same conditions, p -cyanophenol afforded a 70% yield of the desired product 2e ( Table 2 , entry 6), confirming that the C–O coupling catalysis can be extended to other phenols. The catalytic reactivity could be additionally extended to C–C couplings, as demonstrated by the 68% yield of 2h coupling product obtained by the catalysis with L 1 –I , malononitrile (10 equiv. ), 10 mol% of AgOTf and 10 mol% of PPh 3 ( Table 2 , entry 8). On the other hand, when the substrate L 1 –I is replaced by L 1 –Br , containing a stronger C aryl –halide bond, the yields of the catalytic reactions were reduced to a maximum of 21% of 2d ( Table 2 , entry 11). As expected, these low yields were clearly enhanced by using 2 equiv. of Tl(OTf) as additive under the same catalytic conditions, obtaining a 43% yield of 2d ( Table 2 , entry 12). More importantly, the implication of the aryl-Ag(III) species as competent catalytic intermediate species was demonstrated by performing the catalytic coupling of L 1 –I and p -nitrophenol using 10 mol% of 1 ClO4 and 10 mol% of PPh 3 under the standard catalysis conditions ( Table 2 , entry 9), to find that the same yield as in the catalysis with 10 mol% AgOTf was finally obtained. 1 H-NMR monitoring of the catalytic reaction corroborated the formation of the aryl-Ag(III) (4%) as active species during the course of the reaction (see Supplementary Fig. 18 ). A key aspect to rationalize the observed catalysis consists of the ability to prevent the precipitation of AgI so that catalytic turnover becomes possible. We observed that the large excess of p X-phenol used in the catalysis delayed the precipitation of AgI (for turbidity monitoring experiments see Supplementary Fig. 19 ) and might form coordination complexes with silver(I) (by HRMS, see Supplementary Figs 20 and 21 ), thus preventing the precipitation of AgI. On the other hand, we realized that excess of iodide caused the formation of monoanionic AgI 2 − in solution (by HRMS, see Supplementary Figs 22 and 23 ) and completely quenched the precipitation of AgI ( Supplementary Fig. 19 ) [40] , [41] . To further substantiate that monoanionic dihalide silver(I) species can participate in the cross-coupling reactions described, we attempted a halide exchange catalysis starting with L 1 –I model substrate, 10 mol% AgOTf and 10 equiv. of n Bu 4 NBr. The substrate was quantitatively converted to L 1 –Br in 24 h without any sign of precipitation during the catalytic reaction (see Fig. 4 ). In addition, AgI 2 − , AgBrI − and AgBr 2 − monoanionic species were detected by HRMS ( Supplementary Fig. 24 ). In addition, the slight beneficial effect of PPh 3 might be related to the formation of monocationic [Ag(PPh 3 ) 2 ] + species, which was detected by HRMS ( Supplementary Fig. 25 ) under the catalytic conditions of entry 3, Table 2 , thus also contributing to prevent the precipitation of silver(I) out of the solution. 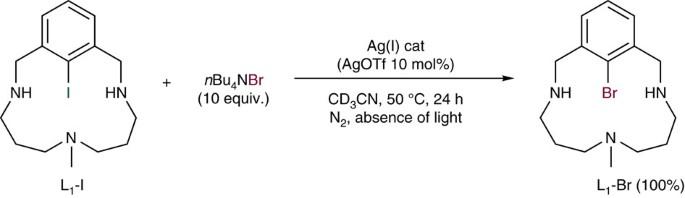Figure 4: Silver(I)-catalysed bromination of model aryl iodide substrate. Conditions: [L1–I]=5 mM, [nBu4NBr]=50 mM, [AgOTf]=0.5 mM, 3 ml CD3CN, 50 °C; yield calculated by1H-NMR spectroscopy using 1,3,5-trimethoxybenzene as internal standard. Figure 4: Silver(I)-catalysed bromination of model aryl iodide substrate. Conditions: [ L 1 –I ]=5 mM, [nBu 4 NBr]=50 mM, [AgOTf]=0.5 mM, 3 ml CD 3 CN, 50 °C; yield calculated by 1 H-NMR spectroscopy using 1,3,5-trimethoxybenzene as internal standard. Full size image Further investigations were performed to evaluate the possibility that coupling reactions involve an initial single electron transfer (SET) step. Cyclic voltammetry experiments indicate that the Ag(III)/Ag(II) reduction is electrochemically irreversible and has a reduction potential of −0.6 V versus non-aqueous Ag/AgNO 3 reference electrode ( Supplementary Fig. 26 ). As the oxidation potential of p- nitrophenol is E 0 ox >1.3 V (versus Ag/AgNO 3 ) [42] , [43] , SET from the latter to the Ag(III) complex is highly disfavoured (1.9 V difference, Δ G 0 =43.8 kcal·mol −1 ). Moreover, DFT calculation of the first SET from p -nitrophenol to Ag(III) to afford a phenoxyl radical and aryl-Ag(II) is thermodynamically endergonic (Δ G =41.6 kcal·mol −1 , in close agreement to the value deduced from cyclic voltammetry data, see Supplementary Fig. 27 for computed reaction profile), thus clearly disproving SET in our mechanism. In addition, the DFT-calculated pathway for the reductive elimination of aryl-Ag(III)-( p NO 2 -phenolate) species to afford the p NO 2 -Ph-O-Aryl coupling product and Ag(I) provides theoretical evidence for a single transition state with a small energy barrier of 16.6 kcal·mol −1 ( Supplementary Fig. 28 ). Furthermore, the activation parameters for the reaction of 1 ClO4 with p -cyanophenol could be determined by ultraviolet–visible monitoring of the decay of the aryl-Ag(III) providing a Δ G ≠ (298K)=24.5±0.6 kcal·mol −1 (for the Eyring plot of the reaction see Supplementary Fig. 29 ). This value is in reasonable agreement with that computed for our proposal of a two-electron reductive elimination process ( Supplementary Fig. 28 ). Therefore, a general two-electron-based Ag(I)/Ag(III) mechanistic proposal that accommodates all the experimental data collected in this study is depicted in Fig. 5 . 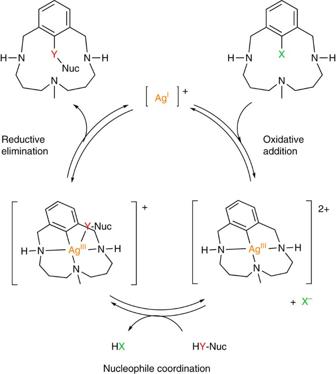Figure 5: Mechanistic proposal operating via aryl-Ag(III) species. General proposed mechanism of Ag(I)-catalysed cross-coupling reactions through the intermediacy of aryl-Ag(III) complexes using model aryl halide substrates. Figure 5: Mechanistic proposal operating via aryl-Ag(III) species. General proposed mechanism of Ag(I)-catalysed cross-coupling reactions through the intermediacy of aryl-Ag(III) complexes using model aryl halide substrates. Full size image In summary, we have demonstrated that the canonical one-electron redox reactivity of silver can be surpassed. The fundamental oxidative addition and reductive elimination steps involved in Ag(I)/Ag(III) redox chemistry have been clarified and this provides a solid mechanistic understanding of a completely new reactivity for silver. These results represent a breakthrough in the fundamental understanding of silver’s redox chemistry, and opens potential new avenues for designing Ag-catalysed synthetic tools in organic synthesis, in a direct parallel to the well-known Pd(0)/Pd(II) and Cu(I)/Cu(III) catalysis [20] . General materials and methods Reagents and solvents used were commercially available reagent quality unless indicated otherwise. Solvents were purchased from SDS-Carlo Erba and Scharlab and were purified and dried by passing through an activated alumina purification system (MBraun, SPS-800). Preparation and handling of air-sensitive materials were carried out in a N 2 drybox (JACOMEX) with O 2 and H 2 O concentrations <1 p.p.m. NMR data were collected on a BRUKER 400 or 300 AVANCE spectrometer (BRUKER or AVANCE) in the corresponding deuterated solvent (CDCl 3 or CD 3 CN) and calibrated relative to an external 1 H reference (1,3,5-trimethoxybenzene). Conventional 1D 1 H, 13 C{ 1 H}, 19 F{ 1 H}, 31 P{ 1 H} and two-dimensional (2D) 1 H– 1 H correlation spectroscopy (COSY), 1 H– 1 H nuclear Överhauser enhancement spectroscopy (NOESY), 1 H– 13 C heteronuclear single quantum coherence (HSQC) experiments were recorded under routine conditions. 109 Ag NMR experiments were collected in a broadband fluorine observation (BBFO) probe using a sample of 1 M AgNO 3 as an external chemical shift reference and for pulse and frequency calibration. The 1D 1 H{ 109 Ag} spectrum was recorded with the pulse programme zgig (included in the TOPSPIN v2.1 software package), using a recycle delay of 1 s. 2D 1 H- 109 Ag HMBC spectrum was collected using the standard pulse programme hmbcgpndqf, with a defocusing period of 65 ms (optimized to 8 Hz) and using a relative gradient ratio of G1:G2:G3=70:30:44.7, which was established as a function of the gyromagnetic ratios between 1 H and 109 Ag nuclei. Equivalent 2D 1 H- 109 Ag HSQMBC-IPAP and HSQMBC-COSY-IPAP experiments were acquired using the pulse schemes and general acquisition conditions described in the literature [44] . The relevant parameters concerning Ag-NMR studies are listed below [45] : 109 Ag; spin ½, natural abundance 51.82%, gyromagnetic moment/γ -1.087·10 7 radT −1 s −1 , relative receptivity 0.197 107 Ag; spin ½, natural abundance 48.18%, gyromagnetic moment/γ -1.250·10 7 radT −1 s −1 , relative receptivity 0.279. HRMS were recorded on a Bruker MicrOTOF-Q IITM instrument (Bruker) using electrospray ionization (ESI) or Cryospray ionization sources at Serveis Tècnics de Recercaof the University of Girona. C, H, N elemental analyses were performed on a ThermoFinnigan Flash-EA1112 analyzer. Electrochemical measurements of 1 ClO4 were carried out on a Workstation CH-600E series (CH Instruments). The compound (1 mM) was dissolved in a degassed solution of nBu 4 NPF 6 (0.1 M) in CH 3 CN. The measurements were performed under constant flux of N 2 employing a three-electrode setup: 3-mm-diameter Teflon-shrouded glassy carbon working electrode, a Pt wire auxiliary electrode and a non-aqueous Ag/AgNO 3 reference electrode (purchased from CH Instruments). All potential values are reported with respect to non-aqueous Ag/AgNO 3 reference electrode. Turbidity measurements to monitor the precipitation of silver as AgI in the presence and absence of p -nitrophenol were performed by multiple light scattering techniques on a Turbiscan LAB instrument. All reagents used for stoichiometric and catalytic experiments were weighed in a precision balance (legibility 0.01 mg) and then brought in an inert-atmosphere glove box to perform the reactions. Synthesis and characterization of complex [Ag III (L 1 )](ClO 4 ) 2 (1 ClO4 ) Complex [ Ag III (L 1 )](ClO 4 ) 2 was prepared by dropwise addition of a solution of AgClO 4 (2 equiv.) in CH 3 CN to a vigorously stirred solution of L 1 –Br in CH 3 CN under inert atmosphere. After few seconds, the solution became cloudy turning bright yellow and a precipitate appeared. After 2 h, the reaction mixture is centrifuged, filtered through Celite and then through an Acrodisc filtre. Slow diethyl ether diffusion over the resulting solution afforded yellow crystals of the desired complex. [Ag III (L 1 )](ClO 4 ) 2 (1 ClO4 ): (68% yield) 1 H-NMR (400 MHz, CD 3 CN, 25 °C) δ , p.p.m. : 7.27 (t, 1H, J =7.58 Hz, H a ), 7.06 (d, 2H, J =7.52 Hz, H m ), 6.66 (bb, 2H, NH ), 4.86 (dd, J =16.32 Hz, 3 J(H c - 109 Ag)=11.5 Hz, 2H, H c ), 4.73 (d, J =16.2 Hz, 3 J(H d - 109 Ag)=1.5 Hz, 2H, H d ), 3.44–3.37 (m, 2H, H e or H f ), 3.33–3.27 (m, 2H, H e or H f ), 3.15–3.08 (m, 2H, H i or H j ), 2.81–2.78 (m, 2H, H i or H j ), 2.64 (s, 3H, H k ), 2.20–2.11 (m, 4H, H g or H h ). 13 C-NMR (100 MHz, CD 3 CN, 25 °C) δ , p.p.m. : 186.47 (dd, JC- 107 Ag, JC- 109 Ag =32.60 Hz, 36.72 Hz), 147.90 (C 2 ), 129.65 (C 4 ), 123.19 (C 3 ), 65.35 (C 5 ), 59.35 (C 6 ), 53.42 (C 8 ), 42.55 (C 9 ), 25.58 (C 7 ); 109 Ag NMR (18.62 MHz, CD 3 CN, 25 °C, extracted from the indirect dimension of a 1 H- 109 Ag HMBC spectrum, and taking a sample of 1 M AgNO 3 in D 2 O as a external reference) δ , 2,127 p.p.m. HRMS electrospray ionization-time of flight (ESI-TOF), ( m/z ) calculated for [C 15 H 24 AgClN 3 O 4 ] + , [Ag III ( L 1 )](ClO 4 ), 454.0484, found: 454.0495. Ultraviolet–visible (CH 3 CN): λ max ( ∈ )=390 nm (sh, 540). For the computed structure and spectroscopic and electrochemical data for the characterization of 1 ClO4 see Supplementary Figs 1–10 and Supplementary Fig. 26 . Oxidative addition over L 1 –Cl and L 1 –Br A sample of the L 1 – X ( X =Br, Cl) model substrate (25.4 mg for L 1 –Cl , 29.4 mg for L 1 –Br , 0.090 mmol) and 1,3,5-trimethoxybenzene as internal standard were dissolved in CH 3 CN (0.6 ml). A portion of this solution (0.1 ml) was loaded into an amber vial containing 0.5–2 equiv. of the Ag (I) salt (AgOTf) and 0–10 equiv. of the corresponding additive (NaOTf or TlOTf; Supplementary Table 1 ). The mixture was subsequently diluted with 0.9 ml of CH 3 CN and the vial was sealed with a screw-cap. The mixture was allowed to react for 2 h at room temperature. After that time, the reaction mixture is centrifuged, filtered through Celite and then through an Acrodisc filtre. The resulting solution was evaporated and dried under vacuum. The crude mixture was then redissolved in 0.5 ml of CD 3 CN and transferred to an amber NMR tube and analysed by 1 H-NMR. Final concentrations: [L 1 -X] =15 mM, [Ag I salt]=7.5–30 mM, [additive]=0–150 mM. Reaction yields were obtained by integration of the 1 H-NMR spectra of the crude reaction mixtures relative to 1,3,5-trimethoxybenzene as internal standard (5 mM in CD 3 CN; see Supplementary Table 1 ). Synthesis and characterization of C–N, C–O, C–S and C–C coupling products A sample of the aryl-Ag(III) complex 1 ClO4 (16.3 mg, 0.029 mmol) was dissolved in CD 3 CN (2.1 ml) and 0.2 ml of a solution of 1,3,5-trimethoxybenzene was added as internal standard. A portion of this solution (0.6 ml) was loaded into an amber NMR tube, and 2–10 equiv. of the corresponding nucleophile was added to the tube (0.1 ml, 0.168–0.84 M). Final concentrations: [ 1 ClO4 ]=12 mM and [Nuc]=24–120 mM. The tube was sealed with a septum, and the reaction was allowed to proceed at the corresponding temperature monitoring it by 1 H-NMR spectroscopy until completion. 1 H, 13 C, COSY, NOESY, 1 H– 13 C HSQC NMR spectra and HRMS analysis were obtained without isolation of the C-Nuc coupling product. Spectra corresponding to the monoprotonated form of the products are labelled with HClO 4 . Reaction yields were obtained by integration of the 1 H-NMR spectra of the crude reaction mixtures relative to the internal standard. Synthesis and characterization of the coupling products of boronic acids and 1 ClO4 A sample of the aryl-Ag(III) complex 1 ClO4 (13.3 mg, 0.024 mmol) was dissolved in CD 3 CN (0.9 ml) and 0.1 ml of a solution of 1,3,5-trimethoxybenzene was added as internal standard. A portion of this solution (0.35 ml) was loaded into an amber NMR tube, and 5 equiv. of the corresponding arylboronic acid in CD 3 OD was added to the tube (0.35 ml, 0.12 M). Final concentrations: [ 1 ClO4 ]=12 mM and [arylboronic acid]=60 mM. The tube was sealed with a septum, the reaction was allowed to proceed at 50 °C and was monitored by 1 H-NMR spectroscopy until completion. 1 H, 13 C, COSY, NOESY, 1 H– 13 C HSQC NMR spectra and HRMS analysis were obtained without isolation of the C-Nuc coupling product. Reaction yields were obtained by integration of the 1 H-NMR spectra of the crude reaction mixtures relative to the internal standard. Halogenation of complex 1 ClO4 A sample of the aryl-Ag(III) complex 1 ClO4 (15.5 mg, 0.028 mmol) was dissolved in CD 3 CN (2 ml) and 0.2 ml of a solution of 1,3,5-trimethoxybenzene was added as internal standard. A portion of this solution (0.6 ml) was loaded into an amber NMR tube, and 2 equiv. of the corresponding tetrabutylammonium halide was added to the tube (0.1 ml, 0.168 M). Final concentrations: [ 1 ClO4 ]=12 mM and [ n Bu 4 N X ]=24 mM ( X =Cl, Br, I). Upon addition of the halides, the solution rapidly turns deep orange, indicating some degree of deprotonation of the complex. The tube was sealed with a septum, and the reaction was allowed to proceed at the corresponding temperature and was monitored by 1 H-NMR spectroscopy until completion. 1 H-NMR and HRMS analysis were obtained without isolation of the C–X coupling product. Reaction yields were obtained by integration of the 1 H-NMR spectra of the crude reaction mixtures relative to the internal standard. The characterization of the halogenation products ( L 1 –Cl , L 1 –Br and L 1 –I ) has been achieved by direct comparison with authentic samples synthesized independently [18] , [39] . Fluorination of complex 1 ClO4 A sample of the aryl-Ag(III) complex 1 ClO4 (15.5 mg, 0.028 mmol) was dissolved in CD 3 CN (2 ml) and 0.2 ml of a solution of 1,3,5-trimethoxybenzene was added as internal standard. A portion of this solution (0.6 ml) was loaded into an amber vial, and 2 equiv. of n Bu 4 NF·3H 2 O was added to the tube (0.1 ml, 0.168 M). Final concentrations: [ 1 ClO4 ]=12 mM and [F − ]=24 mM. Upon addition of the fluoride source, the solution rapidly turns deep orange, indicating some degree of deprotonation of the complex. The vial was sealed with a screw-cap and the reaction was allowed to proceed at 40 °C under vigorous stirring. After 24 h of reaction, the crude was centrifuged to remove the black solids generated during the reaction. The resulting solution was evaporated under vacuum and the solids obtained were dried under vacuum for several hours. 1 H-NMR yield of the L 1 –F coupling product was obtained in CD 3 CN and calculated using 1,3,5-trimethoxybenzene as internal standard. 1 H-NMR, 19 F-NMR and HRMS analysis were obtained without isolation of the C–F coupling product. For spectroscopic data for the characterization of the coupling products and its description, see Supplementary Figs 30–106 and Supplementary Methods . Catalytic experiments Stock solutions of L 1 – X /1,3,5-trimethoxybenzene (30/10 mM; x =I, Br), AgOTf/ligand (7.5–15/0–37.5 mM) and of the corresponding nucleophile (0.065–0.13 M) were prepared in CD 3 CN in the glove box. An amber vial was loaded with 0.2 ml of the AgOTf/ligand stock solution and subsequently 2.3 ml of the nucleophile stock solution and 0.5 ml of the L 1 –X /1,3,5-trimethoxybenzene stock solution were added. The vial was sealed with a screw-cap and allowed to react at 50 °C for 24 h. Final concentrations: [ L 1 –X ]=5 mM, [AgOTf]=0.5–1 mM, [ligand]=0–2.5 mM, [Nuc]=0.05–0.1 M. When the reaction time is finished, the crude was transferred to an amber NMR tube and analysed by 1 H-NMR. Reaction yields were obtained by integration of the 1 H-NMR spectra of the crude reaction mixtures relative to 1,3,5-trimethoxybenbenzene as internal standard ( Table 2 main text and Supplementary Table 2 ). The product obtained in the reaction crude was identified by ESI-TOF spectroscopy. See Supplementary Methods section for additional experimental procedures not cited in this part. Crystallographic characterization of [Ag III (L 1 )](ClO 4 ) 2 (1 ClO4 ) Crystals of complex 1 ClO4 were grown from slow diffusion of diethyl ether in a CH 3 CN solution of the compound. All of them were used for low temperature (150(10) K) X-ray structure determination. The measurement was carried out on a Agilent Supernova diffractometer equipped with a 135-mm Atlas detector, and using graphite-monochromated Mo K α radiation ((λ=0.71073 Å) from an X-ray Tube. Programme used for data collection and reduction, CrysAlis pro. Structure solution and refinement were done using SHELXTL Version 6.14 (Bruker, AXS 2000–2003). The structure was solved by direct methods and refined by full-matrix least-squares methods on F 2 . The non-hydrogen atoms were refined anisotropically. The H-atoms were placed in geometrically optimized positions and forced to ride on the atom to which they are attached, except N–H hydrogens, which were located in the difference Fourier map and refined without constrains. See Supplementary Table 3 for crystallographic data and structure refinement of 1 ClO4 . Computational details The Cartesian coordinates of the X-ray diffraction structure of 1 ClO4 have been used as starting point in DFT optimizations. An explicit molecule of CH 3 CN, which is coordinated in the L 1 – X –Ag(I) or L 5 – X –Ag(I) complexes ( X =F, Cl, Br, I), has been included in all DFT calculations. All the calculations were carried out using the Gaussian09 programme package [46] . The DFT-B3LYP hybrid exchange-correlation functional [47] , [48] , [49] has been employed to model the silver molecular systems. Geometry optimizations were performed with no symmetry restrictions, using the Stuttgart/Dresden (SSD) core pseudopotential pseudopotential and basis set [50] on the heavier atoms (I, Ag) and the 6-311+G** basis set on all the other atoms. The acetonitrile solvation and London dispersion effects were included in energy and geometry optimization calculations through the solvation model including the role of density (SMD) polarizable continuum model [51] and the B3LYP-D 2 correction [52] . See Supplementary Figs 17 and 18 , 26 and 27 and Supplementary Table 4 . Vibrational frequency calculations based on analytical second derivatives to obtain the enthalpy and entropy corrections ( T =298.15 K) were performed at the same level of theory. The nature of stationary points was also established in solvent-phase, where minima have no imaginary frequencies and transition states have only one. The free energy of the proton was computed as: where is the gas-phase free energy (-6.3 kcal·mol −1 ) [53] and its experimental solvation free energy in acetonitrile (−260.2 kcal·mol −1 ). The term Δ G * represents the free energy change associated with the conversion from a standard-state of 1 M in the aqueous phase and 1 atm in gas phase, to 1 M in both phases. Its value is 1.9 kcal·mol −1 at 298.15 K. How to cite this article: Font, M. et al. Direct observation of two-electron Ag(I)/Ag(III) redox cycles in coupling catalysis. Nat. Commun. 5:4373 doi: 10.1038/ncomms5373 (2014).